Male water striders attract predators to intimidate females into copulation Despite recent advances in our understanding of sexual conflict and antagonistic coevolution between sexes, the role of interspecific interactions, such as predation, in these evolutionary processes remains unclear. In this paper, we present a new male mating strategy whereby a male water strider Gerris gracilicornis intimidates a female by directly attracting predators as long as she does not accept the male's coercive copulation attempt. We argue that this male strategy is a counteradaptation to the evolution of the female morphological shield protecting her genitalia from coercive intromission by water strider males. The G. gracilicornis mating system clearly represents an effect expected from models of the coevolutionary arms race between sexes, whereby one sex causes a decrease in the fitness component of the other sex. Moreover, our study demonstrates a crucial role that interspecific interactions such as predation can have in the antagonistic coevolution between sexes. Predation risk is a powerful factor in the evolution of courtship [1] , [2] , [3] , but its role has not been fully explored. When courting males attract females with visual or acoustic signals that are also conspicuous to predators, the risk of predation usually increases more for the courting males than for the females that respond to these signals. Hence, the evolution of male courtship signals is usually thought to reflect a trade-off between selection to be conspicuous and attract mates and selection to be less conspicuous to avoid predation [4] , [5] . However, in some species, females experience an elevated risk of predation when they search for mates among males that court at relatively safe locations. This can favour the use of conspicuous courtship signals by courting males that help females orient quickly and safely to males and thereby reduce the females' exposure to predators [6] , [7] . In the water strider species of the family Gerridae, the interest of a male is to mate frequently, whereas the interest of a female is to decrease the frequency of copulation [8] . We recently described morphological and behavioural adaptations to this evolutionary conflict in Gerris gracilicornis [9] , [10] . Females of this species evolved a morphological shield over their vulvar opening, preventing mounted males from coercive intromission. Males can achieve copulation only if the female exposes her genitalia. Females do this only in response to water surface vibration signals produced by males [9] . Predatory aquatic insects or fishes are attuned to these vibrations and often approach water striders from below the water surface [11] . A water strider male in a typical mounting position, on top of a floating female, is at a lower risk of predation than is a female during predator attacks on the male–female tandem [12] , [13] , [14] . Therefore, if males mounted on females reveal their location to predators by producing ripple signals [9] , they would increase the risk of predation to the females on which they are mounted rather than to themselves. Here, we test the hypothesis that the ripple signals given off by G. gracilicornis males may have evolved because they increase predation risk to non-responsive females, and because attraction of predators to females that are reluctant to mate when they are mounted by signalling males may decrease their chances of survival compared with females that copulate quickly. We demonstrate that courtship signalling by males attracts predators, which attack females rather than males. We further show that, in response to increased predation risk, females permit copulation sooner, prompting males to terminate signalling more quickly. We also show that, in response to predators, males do not decrease, and large males even increase, their leg tapping movements, which produce the predator-attracting signals. Thus, G. gracilicornis males perform a novel male mating strategy (intimidating courtship) whereby males manipulate the environment to affect the behaviour of predators so as to increase female-biased predation risk, which induces females to expose their genitalia for copulation more quickly. Behaviour of predators We determined whether male signals increase predation risk to G. gracilicornis females. Immediately after detecting water surface vibrations, notonectid predators (Hemiptera, Notonectidae, Notonecta triguttata ) in experimental containers quickly turned their heads and moved towards the source of the signals ( Supplementary Movie 1 ). In Y-maze tests ( Fig. 1a ), notonectids were attracted to the arm with the mating pair having a signal-producing male, rather than to the arm having a silent male ( Fig. 1b , n =17, G =23.5, P <0.001), but they showed no preference when each arm of the Y-maze box had a pair with a signalling male ( Fig. 1c ; n =11, G =0.829, P =0.363). Thus, precopulatory pairs, in which mounted males produce signals, are detected more easily by predators. In addition, all females rather than males ( G =18.0, n =13, P <0.001) in 13 mating pairs subjected to predator attacks (in a separate experiment) were captured by the attacking notonectids, suggesting that predator-attracting ripple signals increase the risk of predation to females rather than to males. 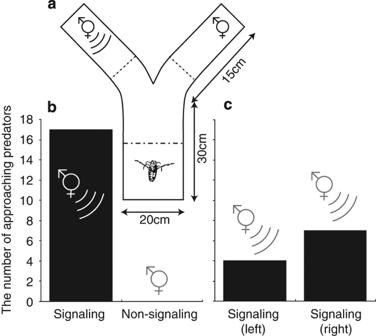Figure 1: Effect of male ripple signals on predator behaviour. (a) Y-maze container used in experiments with predators. (b) Frequency of predator approaches to a pair with a male producing ripple signals (a signalling pair) or a pair with the non-signalling male (a non-signalling pair, postintromission). (c) Frequency of predator approaches to signalling pairs in the arms of the Y-maze. If a predator crossed the arbitrarily set line in an arm (dotted lines), it was scored as entering the arm. Figure 1: Effect of male ripple signals on predator behaviour. ( a ) Y-maze container used in experiments with predators. ( b ) Frequency of predator approaches to a pair with a male producing ripple signals (a signalling pair) or a pair with the non-signalling male (a non-signalling pair, postintromission). ( c ) Frequency of predator approaches to signalling pairs in the arms of the Y-maze. If a predator crossed the arbitrarily set line in an arm (dotted lines), it was scored as entering the arm. Full size image Behaviour of females We asked whether females respond to male signals in a way that reduces the female's risk of predation. A female could cause a male to stop producing predator-attracting vibratory signals by protruding her genitalia. This allows a male to initiate intromission, after which he stops the signalling entirely [9] . In an experiment, we repeatedly tested each female in four treatments in the same order (Control, Predators, Bar, Bar & Predators explained in Methods section) to determine whether females' latency to protrude genitalia decreases from normal (Control) to low immediately after she has experienced predatory attacks (Predators). We then determined whether experimental reduction of the mounted male's ability to produce ripple signals (by using a 'w-bar' glued across the females back [9] ) decreases the female's genital protrusion response to predators (compare Bar and Bar & Predators; Fig. 2 ). In the Methods section, we present details and justification of the fixed-order design, and in Supplementary Table S1 , we present results of parametric analyses (which may be less reliable because the variables did not conform to the parametric statistics' assumptions). 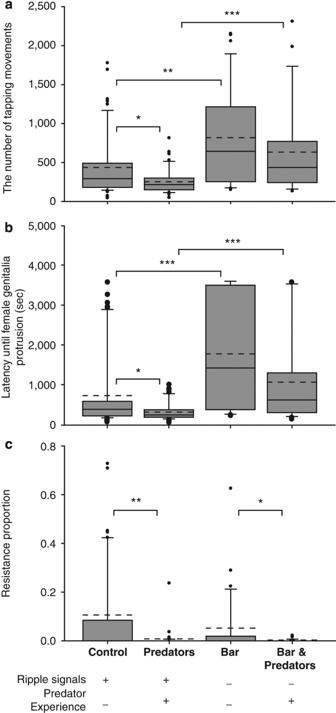Figure 2: Effects of predator attacks and ripple signals produced by males on females. Mating behaviour is expressed as (a) the total number of tapping movements by males during latency until protrusion; (b) latency until genitalia protrusion; and (c) the proportion of latency until protrusion spent by the female in active resistance behaviour. Boxes indicate the 25 and 75% quartiles. Median is marked as a solid line and mean as a dotted line. Outliers are black dots outside the error bars that cut off the lower and upper 10% of the distribution. Asterisks denote significant differences (*P<0.05; **P<0.01; ***P<0.001). Figure 2: Effects of predator attacks and ripple signals produced by males on females. Mating behaviour is expressed as ( a ) the total number of tapping movements by males during latency until protrusion; ( b ) latency until genitalia protrusion; and ( c ) the proportion of latency until protrusion spent by the female in active resistance behaviour. Boxes indicate the 25 and 75% quartiles. Median is marked as a solid line and mean as a dotted line. Outliers are black dots outside the error bars that cut off the lower and upper 10% of the distribution. Asterisks denote significant differences (* P <0.05; ** P <0.01; *** P <0.001). Full size image Because the mounted male's leg tapping (the number of leg movements per bout and the number of bouts per minute) did not significantly change after the female experienced predatory attacks or after the female was equipped with the w-bar, the total number of leg taps received by the female was determined by the female's latency to genitalia protrusion [9] . Females mounted by males who can reach the water surface with their midlegs (Control and Predators in Fig. 2 ) indeed protruded their genitalia shortly after being mounted, that is, only after a few leg tapping movements by the males, and the number of leg movements decreased in tests conducted immediately after a female experienced a predator ( Fig. 2a , Control versus Predators, Wilcoxon signed-rank test, T =235, Z =2.53, n =41, P =0.011; P b =0.022; P b —sequential Bonferroni-corrected P -value). After the ripples from the leg tapping movements of males were dramatically reduced (Bar or Bar & Predators in Fig. 2 ), and regardless of the female's experience with predators ( Fig. 2a , Bar versus Bar & Predators comparison: T =156, Z =0.79, n =27, P =0.428; P b =0.428), the females protruded their genitalia after receiving more male leg movements than in the respective two earlier treatments ( Fig. 2a , Control versus Bar: T =125, Z =2.77, n =33, P =0.005, P b =0.015; Predators versus Bar & Predators: T =24, Z =3.96, n =27, P <0.001, P b =0.004). The correlated latency until genitalia protrusion showed a similar pattern ( Fig. 2b ); it decreased (Control versus Predators, T =272, Z =2.05, n =41, P =0.039; P b =0.078) in tests conducted immediately after a female experienced predator presence, and the effect of recent predator presence was not significant when production of signals by males was reduced (Bar versus Bar & Predators, T =113, Z =1.59, n =27, P =0.112; P b =0.112). After the production of signals by males was reduced by the w-bar, the latency until genitalia protrusion increased (Control versus Bar, T =94, Z =3.33, n =33, P <0.001, P b =0.003; Predators versus Bar & Predators, T =26.5, Z =3.90, n =27, P <0.001; P b =0.004). When mounted, a female can avoid copulation by not protruding her genitalia and by dislodging or throwing the male off her back. These active resistance behaviours create water surface vibrations detectable by notonectid predators. The proportion of time spent by females in active resistance between mounting and intromission significantly decreased after the females experienced predation attempts ( Fig. 2c , Control versus Predators, n =41, T =22, Z =3.25, P =0.001, P b =0.005), even after courtship signals were reduced with the w-bar ( Fig. 2c , Bar versus Bar & Predators, n =27, T =9, Z =2.35, P =0.019, P b =0.055). Experimental reduction of the male's ability to produce ripples did not reduce the female's active resistance ( Fig. 2c ; Control versus Bar: n =33, T =64, Z =1.25, P =0.212, P b =0.379). Hence, the active resistance, which does not affect the termination of male signalling and results in ripples produced by females, was almost absent after experiencing predation attempts, irrespective of whether the male ripple signals were reduced ( Fig. 2c ). This is different from the latency until genitalia protrusion ( Fig. 2b ), which affects predation risk by controlling the total number of male ripple signals. In summary, the behaviour of these female water striders was consistent with decreasing predation risk through decreasing the amount of surface vibrations originating from the mating pair (either a male or a female). Behaviour of males Finally, we tested the effect of recent experience with predators on the behaviour of males in mating interactions with randomly chosen females who had not experienced predators (details in the Methods section). Predator-experienced males significantly increased the log-transformed latency from the beginning of the test until the first grasping attempt (F 1,22 =80.24, P <0.001), regardless of male size (Size, F 1,22 =3.49, P =0.075; Predator×Size interaction, F 1,22 =1.57, P =0.224), suggesting, as expected, that the presence of a predator made males more cautious ( Fig. 3a ). However, after mounting a female, experience with predators did not affect the log-transformed number of signal bouts per minute produced by large ( t 26 =1.287, P =0.209) or small ( t 16 =−0.393, P =0.699) males (interaction term: F 1,42 =1.23, P =0.274; Fig. 3b ). Furthermore, the log-transformed number of leg movements per bout ( Fig. 3c ; see Han and Jablonski [9] for signal structure description) increased in response to predator treatment for large ( t 26 =−2.508, P =0.019), but not for small ( t 16 =1.209, P =0.244), males (interaction term: F 1,42 =6.263, P =0.016). Hence, it seems that, in response to predators, males did not decrease, with large males even increasing, their leg tapping movements that produce the predator-attracting signals. The male behaviour was consistent with the idea that males actively attract predators to exploit the predation-minimizing behaviour of females. 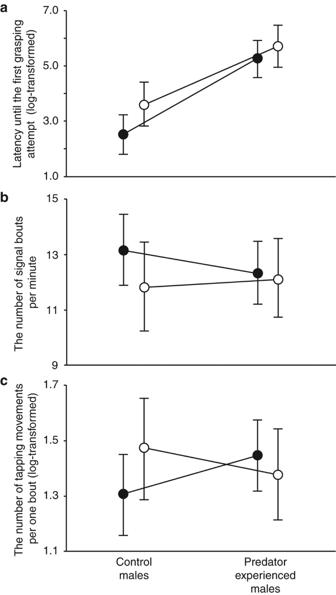Figure 3: Effect of experience with predators and the size of males. Effect was measured as (a) log-transformed latency until the first mate-grasping attempt by a male (13 large and 11 small males) (b) the number of signal bouts per minute (27 large and 17 small males); and (c) the log-transformed number of tapping movements per bout by a male (27 large and 17 small males). Males were categorized as large (closed circles) or small (open circles). Error bars indicate 95% confidence intervals around mean. Figure 3: Effect of experience with predators and the size of males. Effect was measured as ( a ) log-transformed latency until the first mate-grasping attempt by a male (13 large and 11 small males) ( b ) the number of signal bouts per minute (27 large and 17 small males); and ( c ) the log-transformed number of tapping movements per bout by a male (27 large and 17 small males). Males were categorized as large (closed circles) or small (open circles). Error bars indicate 95% confidence intervals around mean. Full size image Postponing the moment of intromission by delaying genitalia protrusion by females and the attempts of mounted males to shorten latency until intromission create conditions necessary for the evolution of this intimidating courtship signalling in G. gracilicornis . These conditions are the outcome of the evolutionary conflict between the interests of males and females to mate more and less frequently, respectively [8] . In many water striders, in which genitalia are exposed and susceptible to coercive copulation, females oppose mating by fighting with males. Because males can be more easily thrown off if their genitalia are not inserted, the conflict between sexes promotes, among others, the evolution of male adaptations to shorten, and female adaptations to prolong, latency until intromission. This antagonistic coevolution has led to female-specific morphological adaptations such as spines and male-specific posterior body shapes in water striders [15] . The use of genitalia protrusion from behind a morphological protective shield by females to fully control intromission has only been reported in G. gracilicornis as an apparent means to completely block forced intromission by males [9] , [10] . Our current results demonstrate that males apparently responded by counterevolution of the conspicuous intimidating signals that attract predators and increase predation risk to females ( Supplementary Movie S1 ). Moreover, it seems that some males may be able to adaptively increase the use of intimidating signals in the presence of predators. Similar male leg tapping movements are also present in Aquarius najas , in which they induce genitalia protrusion in females but do not result in ripple signals [16] . The leg tapping of A. najas represents a hypothetical candidate for the ancestral behavioural trait in the evolutionary sequence leading to the ripple-producing and predator-attracting courtship of G. gracilicornis . Alternatively, the intimidating courtship might have evolved from the already existing ripple signalling system, typically present in water striders in the context of mating and aggression [9] . Regardless of the particular evolutionary scenario, our results indicate that rapid evolution of this new intimidating function of the ripple-producing leg tapping occurred in response to the evolution of the female's genital shield [9] . A male courtship tactic such as this would be expected to become fixed quickly because of the clear benefits to males, the clear fitness costs to females who do not respond to this signal, as well as a dramatic decrease of these costs in females who respond by genitalia protrusion. Generally, the theory [8] , [17] predicts that any potentially harmful (to females) male behaviour evolves when benefits to males (here in terms of increased mating success of the signalling males) are higher than the fitness costs to females who evolve an adaptive response to the male behaviour (here females who respond to the signal). Because the predation risk dramatically decreases if no ripple signals are produced, the costs to such sensitive (responding) females are indeed probably very low, even considering costs of superfluous mating [18] , [19] . Fitness benefits to the ripple-producing males in G. gracilicornis are high because of competition between males for copulation [18] . Ongoing research will provide numerical estimations of these fitness costs and benefits in order to fully understand the evolutionary dynamics of the antagonistic coevolution between sexes in G. gracilicornis . A hypothetical 'mate choice' mechanism may additionally contribute to the female's delay in genitalia protrusion and to the initial evolution of male midleg tapping movements. The energetic leg tapping movements are experienced by a female G. gracilicornis , irrespective of whether the movements result in ripple signals [9] . Similar movements are also present in another species, A. najas , in which they do not result in ripple signals at all [16] . Females of both species protrude their genitalia after a mounted male performs tapping movements with his midlegs. Therefore, a hypothesis that females of these species may use the male tapping leg movements to collect information about a male's quality before deciding whether to protrude her genitalia cannot be rejected. However, the observed significant effect of the bar treatment on female behaviour cannot be explained by the mate choice hypothesis, because these behavioural differences in female acceptance of mating are not associated with significant differences in the leg tapping movements by males between these treatments. Thus, the hypothetical mate choice mechanism cannot fully account for the results of our experiments. We also considered the hypothesis that actual ripples, rather than tapping leg movements, provide some information to females for their mate choice decisions. Because the w-bar drastically decreases the rate of this information transfer, sampling for longer duration (latency until genitalia protrusion and the correlated total number of tapping leg movements by the male) is needed before the female decides to protrude her genitalia. This prediction is also consistent with the 'intimidating courtship hypothesis'. However, the lack of significant difference in female responses when the efficiency of attracting predators is small in the w-bar treatments (Bar versus Bar & Predators), combined with the presence of significant difference when the risk of attracting predators is high (Control versus Predators), indicates that ripple signals, but not leg movements, from males sensitize females to the presence of predators. This is directly predicted from the 'intimidating courtship hypothesis' and not from the 'mate choice hypothesis.' Although we cannot reject or accept the mate choice function of the ripple signals, the patterns of female behavioural responses to all experimental treatments support the intimidation hypothesis, regardless of whether the females extract information about males from their signals. The intimidation hypothesis is further confirmed by the increase in the use of ripple signals by large males in response to the presence of predators, and the lack of effect of predators on small males in this context. We suggest two hypotheses to explain differences between large and small males. If a male in a mating position is at a lower risk during a predator's attack than a single male, and if small males can be more easily thrown off by females, then the small males are at a higher predation risk, especially if they have already attracted predators by producing ripples. Therefore, smaller males may be more reluctant to produce signals if predators are present. We also hypothesize that the strength of intimidating effect on females may be determined by the body size (or body mass) of males. If larger males, with longer midlegs and heavier body, are able to produce stronger ripples (high amplitude), they attract predators from a larger distance (larger surface area) than do small males. Increasing the number of ripples may lead to increased chances of attracting predators for large rather than small males. We predict that, in response to predator presence, large males increase conspicuous signalling to a higher degree than do small ones, because the expected increase in benefits for the male is greater. It is known that males of some species can switch to a different mating strategy in response to female behaviours performed in situations of increased predation risk [20] , [21] . Males in some moth species were suggested to induce antipredatory 'freezing' behaviour in females by imitating vocalizations of predators (bats) to exploit the female's immobility for mating [22] , [23] . Male crabs manipulate female behaviour by modifying the physical environment to provide safe sites for females [6] , [7] . G. gracilicornis males perform a novel male mating strategy, whereby males manipulate the information content of the environment to affect the behaviour of predators so as to increase female-biased predation risk, which induces females to protrude their genitalia for copulation more quickly. The results illustrate how behavioural adaptations to the arms race between sexes may be shaped by predation. Study subjects The experimental specimens G. gracilicornis were collected at Gwanak Mountain near Seoul National University. They were then separated into two rectangular plastic containers (40×50 cm) according to gender, and fed ad libitum with surplus frozen crickets ( Verlarifictorus asperses ) every 2 days. Pieces of floating styrofoam were used as rest sites for the water striders. All animals were individually marked on the thorax with enamel paint. Effect of male signals on predator behaviour A pair of G. gracilicornis , with a male producing courtship signals, and a pair with a non-signalling male (in preintromission and postintromission stage of mating interactions, respectively) were placed in two arms of a Y-shaped container filled with water ( Fig. 1a ). A partition (dotted line of Fig. 1a ) in each arm restricted the pair movements but allowed for the ripple signals produced by the male to travel on the water surface towards the basal arm, where a notonectid predator that had not been fed for 24–72 h was introduced. The predator was isolated in the basal arm by a plastic partition (broken line of Fig. 1a ) for 2 min, after which it was allowed access to the two arms. When the predator crossed an arbitrarily set line in either arm ( Fig. 1a ), it was scored as approaching the water striders in the particular arm. Seventeen notonectids were tested in this experiment, switching the location of the signalling pair between arms for each test. Eleven notonectids were tested in the same setup, but with both arms containing pairs with signalling males. Effect of predator attacks on the mating pair In 13 trials, we watched the attack of one predator on a pair of water striders in an experimental tank (15×15 cm) filled with water. Effects of predators and ripple signals on female behaviour We measured the effect of female experience with predators and the effect of experimental reduction of ripple signals by males on the female by (1) latency until genitalia protrusion (duration in seconds from the moment a male grasped any part of the female's body until the protrusion of female genital segments, which is the final action for successful intromission); and (2) the total number of tapping movements by males during latency until female genitalia protrusion. We regard the latter as a better index of female behaviour that directly affects predation risk to the mating female because the signals are directly attracting predators. The mounted male's leg tapping rate (the number of tapping movements per bout and the number of bouts per minute) did not significantly change after the female experienced predatory attacks (Control versus Predators comparison: Wilcoxon signed-rank test, T =96.5, Z =1.26, n =24, P =0.207 for the number of tapping movements per bout; T =133, Z =0.49, n =24, P =0.627 for the number of bouts per minute), or after the female was equipped with the w-bar (Control versus Bar comparison: T =38.0, Z =0.52, n =14, P =0.600 for the number of tapping movements per bout; T =48, Z =0.28, n =14, P =0.778 for the number of bouts per minute). Therefore, the total number of leg taps received by the female was determined by the female's latency to genitalia protrusion [9] . Given that most males stopped signalling immediately after successful intromission [9] , the two variables were strictly correlated. On some occasions, females did not allow intromission for up to 1 h, in which case, latency until protrusion was recorded as 3,600 s (the number of leg movements was counted until that moment only). We also measured (3) resistance proportion defined as the proportion of latency until genitalia protrusion spent by the female on attempts to get rid of the male. These attempts often produce surface vibrations that can be detected by predatory notonectids. To assess the effect of experience with predators and the effect of ripple signals on female behaviour, we tested each experimental female under four conditions in fixed order. In preliminary trials, water strider behaviour did not differ on 6 consecutive days (latency until genitalia protrusion, Friedman's test: χ 2 =4.05, d.f.=5, n =10, P =0.541; the total number of tapping movements, χ 2 =8.81, d.f.=5, n =10, P =0.117; resistance proportion, χ 2 =4.18, d.f.=5, n =10, P =0.52). We therefore used a fixed order of treatments in the main experiment. The fixed order was also preferred because the experimental manipulation of females is irreversible, and minimized the impact of collection on the local wild population. First, a female was tested in Control treatment before any presentation of predators, followed by three experimental treatments conducted at 1- to 2-day intervals. After the Control treatment, a female was tested in the Predators treatment, that is, after a female experienced attack attempts by notonectid predators just before the trial. After the Predators treatment, each female was equipped with a w-bar across her back, according to the methods by Han and Jablonski [9] . Although the w-shaped bar is attached to the female's thorax, it does not affect the male's leg tapping movements but reduces the production of ripple signals by males by 42% in comparison with females without a bar. The weight of the bar does not significantly affect the female's behaviour [9] . The Bar and Bar & Predators treatments were conducted at the end, because, once the w-bar was attached, it could not be removed without a risk of injuring the females. Each female was tested in the 'Bar' treatment after acclimation to the w-shaped bar for 1 day in a container with other experimental females. Finally, the day after Bar treatment, the female (with w-bar attached) was tested immediately after she experienced predatory attempts from notonectids (Bar & Predators) as in the Predators treatment. Immediately after each test, the experimental individuals were returned to their rearing containers, separated according to sex, where they could interact with others of the same sex in the container and would not encounter predators. This was intended to minimize any effect of previous treatments, especially the effect of predator experience from the Predators treatment on the consecutive Bar treatment. Because the interactions with predators in the Predator treatment lasted for just a few minutes and occurred 16–24 h before the Bar treatment test, during which time the experimental females interacted only with other females, we felt confident that the effect of predator experience in Predators treatment would sufficiently diminish by the time of the Bar treatment. We started with 57 females, but some died or escaped before the trials ended. Thus, the sample sizes are different for different comparisons between treatments. The transparent tank (made of acrylic plate, 15×30 cm) was divided by an opaque partition (5×15 cm; height×length) into two separate containers (15×15 cm) for blocking the transmission of chemical and vibratory signals through the water between the two parts (each part was filled with water up to 4.8–5.0 cm). A second opaque plate (10×15 cm) was located above the first one and could be lifted by the experimenter to allow the water striders, but not the notonectids, to move from one part to another. In each test, a female was introduced into one half and a male into the other half for 3 min, after which the partition was lifted to allow the female to move to the experimental compartment with the male. In the Predators and Bar & Predators treatments, 4–5 notonectid predators were introduced into the compartment with the female. After 10 unsuccessful predator attacks or after one successful grasping by the predator, the female was allowed to escape to the second compartment with a male. Experimenters always interrupted a successful predatory grasping to prevent predators from piercing the cuticle of the water strider with their rostrum. Effects of predators on male behaviour In one experiment, we measured the effect of predators on latency until the first grasping in 24 males. In another experiment, we measured the effect of predators on the number of signals per bout, as well as on the number of signal bouts per minute in 44 males. In 13 preliminary trials, the males' reactions did not differ between two consecutive days (latency: T =40.5, Z =0.439, n =13, P =0.727; number of signals per bout: T =42, Z =0.244, n =13, P =0.807; number of signal bouts per minute: T =42, Z =0.244, n =13, P =0.807). Thus, the effect of predators was measured by comparing the two treatments in fixed order. For the first test, a randomly chosen female was introduced to a male who had not experienced predators (Control treatment). The next day, after being kept with other males in a male-only container without predators, the male was tested again immediately after experiencing predators (Predators treatment). Statistical analyses When original or transformed variables conformed to the assumptions of parametric statistical methods, we used analysis of variance (ANOVA) and t -tests, otherwise we used the non-parametric Wilcoxon signed-ranked test, followed by sequential Bonferroni's correction [24] of the significance level (for n =4 comparisons). In addition, we also applied Friedman ANOVA and parametric ANOVA on log-transformed variables (even though the transformed variables did not conform to the assumptions required for the parametric analysis). Results of the Friedman and parametric ANOVA are shown in the Supplementary Table S1 . For frequencies we used the G -test. Males were divided into two size categories: small (11.9–12.2 mm) and large (12.7–13.4 mm). How to cite this article: Han, C.S. et al . Male water striders attract predators to intimidate females into copulation. Nat. Commun. 1:52 doi: 10.1038/ncomms1051 (2010).